High pressure effects revisited for the cuprate superconductor family with highest critical temperature How to enhance the superconducting critical temperature ( T c ) has been a primary issue since the discovery of superconductivity. The highest T c reported so far is 166 K in HgBa 2 Ca 2 Cu 3 O 8+δ (Hg1223) at high pressure of 23 GPa, as determined with the reduction onset, but not zero, of resistivity. To clarify the possible condition of the real maximum T c , it is worth revisiting the effects of pressure on T c in the highest T c family. Here we report a systematic study of the pressure dependence of T c in HgBa 2 CaCu 2 O 6+δ (Hg1212) and Hg1223 with the doping level from underdoped to overdoped. The T c with zero resistivity is probed with a cubic-anvil-type apparatus that can produce hydrostatic pressures. Variation, not only increase but also decrease, of T c in Hg1212 and Hg1223 with pressure strongly depends on the initial doping levels. In particular, we confirm a maximum T c of 153 K at 22 GPa in slightly underdoped Hg1223. Knowledge of the effects of pressure on superconducting critical temperature ( T c ) is of paramount importance for understanding the mechanism of superconductivity, as exemplified by the latest report on the pressure-induced above-200 K superconductivity [1] . In the conventional superconductors such as MgB 2 , T c decreases with increasing pressure reflecting the decrease of density-of-states at the Fermi level [2] , whereas in some of the unconventional superconductors such as FeSe, T c increases with increasing pressure [3] at least within a certain range of pressure. In the most of high- T c superconductors (HTSCs) with CuO 2 layers, T c increases with pressure in a manner strongly depending on the composition and doping level [4] . Mercury-based HTSCs denoted as the general formula HgBa 2 Ca n −1 Cu n O 2 n +2+δ ( n =1, 2, 3, 4,...) show very high values of T c already at ambient pressure (AP): 95, 127, 134, and 130 K for n =1, 2, 3, and 4, respectively [5] , [6] , [7] . Studies of pressure effects on T c were started just after the discovery of this homologous series, and the maximum values of T c for HgBa 2 CaCu 2 O 6+δ (Hg1212) and HgBa 2 Ca 2 Cu 3 O 8+δ (Hg1223) were reported to be 154 K (ref. 8 ) and 166 K (ref. 9 ) at ∼ 25 GPa, respectively. Gao et al. [8] argued that a universal upward shift in T c was a common feature for all Hg 12( n −1) n . Although these values of T c are commonly accepted, we believe they should be reinvestigated to better understand the effects of high pressures in the light of advances in materials synthesis and high pressure technique; these values of T c were determined from the so-called onset temperature, at which resistivity begins to deviate at a steeper rate from those at higher temperatures with decrease of temperature, whereas the observation of zero resistivity, which literally defines superconductivity, was not attained. Furthermore, in previous studies the pressure above 10 GPa was generated with a diamond-anvil cell [8] , [9] , which does not necessarily ensure the generation of pressures of excellent hydrostatic nature. For a precise study on effects of pressure on zero resistance T c , high-quality hydrostatic pressures are required. To address these issues, we have reinvestigated the effects of pressure on T c in Hg-HTSCs using high-pressure-synthesized dense polycrystalline samples and nearly hydrostatic pressures. Recently, we briefly reported that T c above 150 K could be achieved with zero resistivity in pressurized Hg1223 (ref. 10 ). In the present work, we study the pressure dependence of T c in both Hg1212 and Hg1223 over a wide range of doping level; for Hg1212 a large and critical doping dependence of the pressure effect on T c is revealed, while for Hg1223 the T c with zero resistivity increases monotonously with pressure and reaches a maximal value of 153 K at 22 GPa. 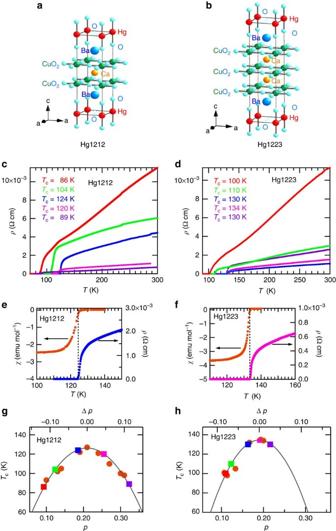Figure 1: Characterization of Hg1212 and Hg1223. (a,b) Crystal structure models of Hg1212 (a) and Hg1223 (b). Red, blue, yellow, green and light blue spheres correspond to Hg, Ba, Ca, Cu and O, respectively. Hashed circle indicates partially occupied oxygen. (c,d) Temperature dependence of resistivity (ρ–T) of Hg1212 (c) and Hg1223 (d) with variousTc. Colour of the curve corresponds to the text colour ofTc. (e,f) Correlation betweenρ–Tand temperature dependence of dc-susceptibility (χ–T) curves exemplified for Hg1212 (Tc=124 K) and Hg1223 (Tc=134 K). (g,h) Estimation of hole concentration (p) for Hg1212 (g) and Hg1223 (h) from a fitting curve (line) using the data in ref.13(solid circle). Squared symbols are data of present study. Colour of the symbol corresponds to the colour of the resistivity in panels of (c,d). Δpstands for the value measured from the optimal doping value at ambient pressure; namely, Δp<0 for underdoped and Δp>0 for overdoped samples. Doping dependence of resistivity at ambient pressure Figure 1a,b show the crystal structures of Hg1212 and Hg1223. These structures offer advantages for investigation of pressure effects. One is the flatness of conductive CuO 2 layer [11] , which would be an important factor for the observed highest T c in HTSCs. This is attributed to coordination of the CuO 2 layer with an elongated Cu–O pyramid, which has a long distance (2.7208(3) Å) between the apical-O (O a ) and Cu owing to a short covalent bond (1.972(3) Å) between Hg and O a (ref. 11 ). Another advantage is that the so-called charge-reservoir block-layer (HgO δ ) is located away from the CuO 2 layer, therefore the extra oxygen least affect local distortion or least cause random potential in CuO 2 layers. Comparison of high pressure effects in Hg1212 and Hg1223 are also interesting, because Hg1212 is composed of only the equivalent two outer CuO 2 layers with an apex-elongated pyramid, while Hg1223 has extra one inner layer of CuO 2 square plane sandwiched by the two outer CuO 2 layers. Figure 1: Characterization of Hg1212 and Hg1223. ( a , b ) Crystal structure models of Hg1212 ( a ) and Hg1223 ( b ). Red, blue, yellow, green and light blue spheres correspond to Hg, Ba, Ca, Cu and O, respectively. Hashed circle indicates partially occupied oxygen. ( c , d ) Temperature dependence of resistivity ( ρ – T ) of Hg1212 ( c ) and Hg1223 ( d ) with various T c . Colour of the curve corresponds to the text colour of T c . ( e , f ) Correlation between ρ – T and temperature dependence of dc-susceptibility ( χ – T ) curves exemplified for Hg1212 ( T c =124 K) and Hg1223 ( T c =134 K). ( g , h ) Estimation of hole concentration ( p ) for Hg1212 ( g ) and Hg1223 ( h ) from a fitting curve (line) using the data in ref. 13 (solid circle). Squared symbols are data of present study. Colour of the symbol corresponds to the colour of the resistivity in panels of ( c , d ). Δ p stands for the value measured from the optimal doping value at ambient pressure; namely, Δ p <0 for underdoped and Δ p >0 for overdoped samples. Full size image The temperature ( T ) dependences of electrical resistivity ( ρ ) in Hg1212 and Hg1223 at AP are shown in Fig. 1c,d . The doping variations in ρ – T curves exhibit common features of in-plane resistivity of HTSC cuprates [12] . The insets show the dc-susceptibility and resistivity of nearly optimally doped samples and confirm that the diamagnetic (Meissner effect) signal starts at the temperature of zero resistivity. This defines the temperature of the superconducting transition, and in the following we adopt such a zero-resistivity temperature as T c . Hole doping level of each sample was estimated from the experimentally established relationship between hole doping and T c reported in ref. 13 , as shown in Fig. 1e,f . Values of T c were determined from the temperature at which the diamagnetic signal begins to appear. We set Δ p = p − p max , where p max gives the maximum T c at AP in the system; by definition, Δ p <0 for the underdoped samples and Δ p >0 for the overdoped samples. Note that the variation in hole concentration of Hg1212 is wider than that of Hg1223. It was difficult to obtain an enough overdoped sample for Hg1223, even after it was annealed under high-pressure oxygen. Doping dependence of resistivity at high pressures The ρ – T curves of Hg1212 and Hg1223 up to 11–13 GPa are shown in Fig. 2 . To facilitate visualization, the resistivities are normalized by the respective values at 270 K, while the absolute values of resistivity reduce by 30–70% from AP to 11–13 GPa. In both Hg1212 and Hg1223, the ρ – T curve in the underdoped (Δ p <0 ) region gradually changes from an upward convex to a straight line, though the degree of the change depends on the initial Δ p values. The superconducting transition itself remains sharp, even at high pressure over 10 GPa. In the positive Δ p (overdoped) region for Hg1212, however, the ρ – T curve is convex downward typical of a normal metal, while the superconducting transition becomes broader with increasing pressure. The origin of the broadened transition under pressures in the overdoped region for Hg1212 is not clear, but such a conspicuous broadening in the resistive transition is also seen for the underdoped region under higher pressures (for example, >15 GPa) where T c turns to decrease with further application of pressure. (We come back to this problem with speculative discussion.) Note that the T c ’s for the Hg1212 samples with Δ p =0.045 (d) and Δ p =0.113 (e) show non-monotonous pressure dependence, namely at first increase and then decrease with increasing pressure. The reason for the rapid increase in T c at relatively low pressure may be ascribed to a pressure-induced structural change, such that the apical oxygen rapidly approaches the CuO 2 layer [14] . Details pressure dependences of T c and d T c /d P in Hg1212 and Hg1223 are shown in the Supplementary Fig. 1 . 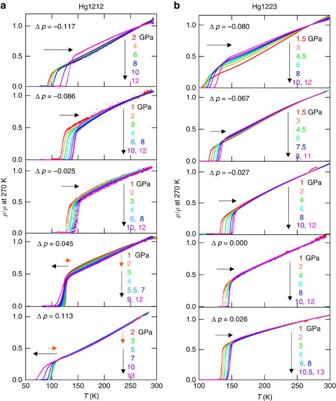Figure 2: Temperature dependence of electrical resistivity of Hg1212 and Hg1223 at high pressures. (a,b) Temperature dependence of electrical resistivity normalized at 270 K for Hg1212 (a) and Hg1223 (b) samples with wide doing levels indicated by Δp. Colour of the curve corresponds to the text colour of pressure. Figure 2: Temperature dependence of electrical resistivity of Hg1212 and Hg1223 at high pressures. ( a , b ) Temperature dependence of electrical resistivity normalized at 270 K for Hg1212 ( a ) and Hg1223 ( b ) samples with wide doing levels indicated by Δ p . Colour of the curve corresponds to the text colour of pressure. 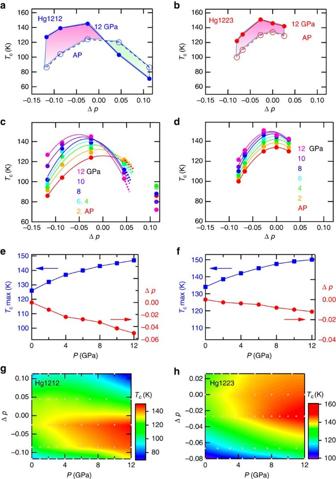Figure 3: Effects of pressure onTcof Hg1212 and 1223. (a,b) Hole doping level (Δp) dependence ofTcin Hg1212 (a) and Hg1223 (b) at ambient pressure (filled circle and solid line) and 12 GPa (open circle and dashed line ). Areas filled with pink and green showTc-increased and—decreased, respectively, with pressure. (c,d) Measured and interpolated valuesof Tcas a function of Δpfor Hg1212 (c) and Hg1223 (d) at high pressures. The parabolic solid lines show the fitting for the constant-pressureTcversus Δpcurves. Colour of the line and circle corresponds to the text colour of the pressure. (e,f) Pressure (P) dependence ofTcmaximum (blue square) and Δp(red circle) that providesTcmaximum for Hg1212 (e) and Hg1223 (f). These values are estimated by the fitting curves of panel (c,d). (g,h)Tccontour maps on pressure doping level (P–Δp) diagram in Hg1212 (e) and Hg1223 (f). A colour bar showsTcvalue in Kelvin. The dots in pale pink correspond to the measured data points. Full size image Figure 3 shows the Δ p dependence of T c in Hg1212 and Hg1223. Figure 3a exemplifies the variation of T c between at AP and 12 GPa in Hg1212. The values of T c in the samples with negative Δ p are increased by more than 30 K with application of pressure up to 12 GPa; notably in the most underdoped (Δ p =−0.113) sample the T c is increased as much as by 41 K. In contrast, the samples with positive Δ p show the pressure-induced reduction of T c . Such a clear reduction of T c with pressure has rarely been reported in HTSC cuprates except for overdoped Tl 2 Ba 2 CuO 6+δ (Tl2201) (ref. 15 ). In Hg1223, on the other hand, T c is simply increased by about 20 K from AP up to 12 GPa in each sample shown in Fig. 3b irrespective of positive and negative value of Δ p , while the pressure effect on T c appears smaller as compared with those for Hg1212 (cf. Supplementary Fig. 1 ). Figure 3: Effects of pressure on T c of Hg1212 and 1223. ( a , b ) Hole doping level (Δ p ) dependence of T c in Hg1212 ( a ) and Hg1223 ( b ) at ambient pressure (filled circle and solid line) and 12 GPa (open circle and dashed line ). Areas filled with pink and green show T c -increased and—decreased, respectively, with pressure. ( c , d ) Measured and interpolated values of T c as a function of Δ p for Hg1212 ( c ) and Hg1223 ( d ) at high pressures. The parabolic solid lines show the fitting for the constant-pressure T c versus Δ p curves. Colour of the line and circle corresponds to the text colour of the pressure. ( e , f ) Pressure ( P ) dependence of T c maximum (blue square) and Δ p (red circle) that provides T c maximum for Hg1212 ( e ) and Hg1223 ( f ). These values are estimated by the fitting curves of panel ( c , d ). ( g , h ) T c contour maps on pressure doping level ( P –Δ p ) diagram in Hg1212 ( e ) and Hg1223 ( f ). A colour bar shows T c value in Kelvin. The dots in pale pink correspond to the measured data points. Full size image Figure 3c,d shows T c values as a function of Δ p at various pressures (at interval of 2 GPa) for Hg1212 and Hg1223, respectively. The parabolic solid lines represent the fitting curves connecting the constant-pressure T c s. This parabolic fitting to the Δ p versus T c dome appears to fail to cover the overdoped region, for example, Δ p =0.113 for Hg1212, yet can work well for the extrapolation to determine the maximal T c and the corresponding Δ p value. From these curves, we obtain the realizable maximal T c and the corresponding Δ p at respective pressure values, as shown in Fig. 3e,f . Those plots show a clear tendency that the maximal T c is attained at lower Δ p and higher pressures. We can also see such correlation in the T c contour maps on the doping–pressure diagram in Fig. 3g,h . All these analyses suggest that the maximal T c under pressures does not always occur at the optimal doping level at AP; the optimal doping giving rise to the highest T c does depend on the pressure value. The possible highest T c is expected at lower doping levels and higher pressures. In practice, however, it was difficult to generate a hydrostatic pressure above 13 GPa in the present pressure load cell with an anvil size of 4 mm side. Resistivity at high pressure over 20 GPa To realize a higher T c , we tried to generate higher pressures using a newly developed anvil of 3 mm side. This enabled us to achieve a nearly hydrostatic pressure up to 22 GPa, which, to the best of our knowledge, would be the highest pressure attained with a cubic-anvil press for resistivity measurements. The detailed procedure and specification for the higher pressure measurement will be reported elsewhere. In this work, we applied pressures of up to 19–22 GPa on four samples; Hg1212 with Δ p =−0.062, and Hg1223 with Δ p =−0.030, −0.052 and −0.095 to explore the possible highest T c s (zero resistance) under realistic hydrostatic pressures. The hole doping levels of these samples should be nearly optimal to enhance T c at around 20 GPa as expected from the results shown in Fig. 3c–h . Effects of pressure on T c for the Hg1212 and the Hg1223 samples are shown in Fig. 4a,b together with T c mid (peak temperature in d ρ /d P curve) and T c onset (temperature for resistivity to start declining towards zero resistivity). Temperature dependences of resistivity are shown in Fig. 4c,d . Those for other samples of Hg1223 are shown in Supplementary Figs 2 and 3 . 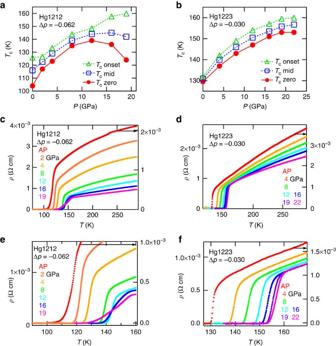Figure 4: Effects of higher pressure on superconductivity in Hg1212 and Hg1223. (a,b) Pressure (P) dependence ofTc zero(zero resistivity),Tc mid(a peak position of dρ/dTin superconducting transition), andTc onset(the resistivity to start to decrease toward zero, as defined by a rising edge in dρ/dT) for Hg1212 (a) and Hg1223 (b). (c,d) Temperature dependence of electrical resistivity (ρ–T) for Hg1212 (c) and Hg1223 (d) Colour of curve corresponds to the text colour of pressure. (e,f) Zoom-up figures of (c–f). Figure 4: Effects of higher pressure on superconductivity in Hg1212 and Hg1223. ( a , b ) Pressure ( P ) dependence of T c zero (zero resistivity), T c mid (a peak position of d ρ/ d T in superconducting transition), and T c onset (the resistivity to start to decrease toward zero, as defined by a rising edge in dρ/d T ) for Hg1212 ( a ) and Hg1223 ( b ). ( c , d ) Temperature dependence of electrical resistivity ( ρ – T ) for Hg1212 ( c ) and Hg1223 ( d ) Colour of curve corresponds to the text colour of pressure. ( e , f ) Zoom-up figures of ( c – f ). Full size image For Hg1212, T c increases up to 12 GPa with the maximum T c of 140 K; above 12 GPa, T c (as defined by zero resistance) decreases although the onset temperature for the resistivity reduction, T c onset , continues to rise. The ρ – T curve is slightly convex upward and the transition width suddenly becomes broad above 12 GPa, as observed in the overdoped samples of Hg1212 (see Fig. 2d,e ). In Hg1223, T c increases up to 22 GPa with the maximum T c of 153 K. Above 19 GPa, T c appears to saturate, although T c mid and T c onset continue to increase, as observed in the former study [10] . Thus, there still remains the possibility of further increasing T c by applying higher pressure to samples with even lower Δ p . In the following, we discuss the possible origins of the observed conspicuous pressure effects on T c . At first, we should note the highly non-monotonous pressure dependence of T c in heavily underdoped samples (for example, Hg1212 with Δ p =−0.11 and Hg1223 with Δ p =−0.08) as shown in Fig. 3g,h and more clearly seen in Supplementary Fig. 3 ; at the first stage of applying pressure, T c does not rise so much, but above 7–8 GPa suddenly increases with the high rate, and then the rate becomes moderate again. This newly found behaviour in T c – P curve for the underdoped region might trace the T c plateau and jump in the T c – p curve, indicative of the charge order or stripe order that is characteristic of the low-doped CuO 2 sheet with the reduced T c (ref. 16 ); such a charge order instability may be removed by pressure above some critical value, for example, 7–8 GPa in the present case. Next, we focus on the difference between the effects for Hg1212 and Hg1223 as exemplified in Fig. 3a,b . The Hg1212 shows clear increase and decrease in T c with application of high pressure in the underdoped and overdoped regime, respectively, while the Hg1223 always shows the increase. One possible reason for this different doping dependence is the fact that only the narrower doping range can be prepared (or the enough overdoped state is difficult to form) for Hg1223 as compared with Hg1212. Another more essential reason is the presence of nonequivalent, that is, inner and outer, CuO 2 layers involved in Hg1223. A former NMR study suggests that the copper valence of the inner layer of HgBa 2 Ca 4 Cu 5 O 12+δ (Hg1245) and TlBa 2 Ca 3 Cu 4 O 10+δ (Tl1234) are lower than those of the outer layer [17] . Redistribution of hole carriers is likely induced among the inner and outer CuO 2 sheets in Hg1223 by applying pressure, which makes the mechanism of pressure-induced T c -change in Hg1223 more elusive than in Hg1212 where the hole-dopable unit is restricted to the crystallographically equivalent CuO 2 sheets with the Cu–O pyramidal coordination. Thus the steeper increase (decrease) of T c with pressure in an underdoped (overdoped) regime should be viewed as the intrinsic feature of the CuO 2 sheets. From the analyses shown in Fig. 3 , in particular for Hg1212, we obtained the result that T c maximum can be realized when starting from an underdoped sample rather than starting from an optimally doped sample. The initial doping level that provides the maximum T c depends on the pressure value, as indicated in Fig. 3e,f . The steep increase and then decrease of T c with pressure as seen in the underdoped (Δ p =–0.062) Hg1212 ( Fig. 4a ) indicates the empirical tendency that application of hydrostatic pressure effectively drives the system toward the overdoping regime; in this particular compound, for example, T c (zero resistance) tends to decrease as the pressure exceeds 12 GPa, as if the compound were placed in the overdoped state (see Fig. 4a ). Furthermore, being characteristic of the overdoped Hg1212 samples ( Fig. 2e ), the superconducting resistive transition becomes broadened in temperature, as manifested by a large discrepancy between T c onset and T c (zero resistance) in the P =16 and 19 GPa data of Fig. 4a . In particular, the high pressure (19 GPa) value of T c onset for Hg1212 reaches 160 K as high as in the case of Hg1223 ( Fig. 4b ). This is the feature commonly observed in previous high-pressure studies [8] , [9] on this highest T c superconductor family. The origin of this broadening of the resistive transition with higher T c onset but lower T c (zero resistance) in the effectively pressure-induced overdoping regime is still not clear; it is hardly ascribable to the pressure inhomogeneity at least in the present experiment, since the superconducting transition under around 20 GPa for Hg1223 (see Fig. 4d ) remains as sharp as at lower pressures. We speculate that the pressure-driven overdoped state may show the tendency of some intrinsic electronic phase separation into the higher T c (>160 K) filaments or embryos and the lower T c (<160 K) state above 20 GPa; however, this issue remains as an important subject of future study. Sample preparation at high pressure The polycrystalline samples of Hg1212 and Hg1223 were synthesized with a cubic–anvil-type high-pressure apparatus (180 ton press, TRY Eng. Co.). Mixtures of HgO, BaO 2 CaO, and CuO/Cu, or mixtures of HgO and the precursor (prepared from BaCO 3 , CaO and CuO at 950 °C in a flowing high-purity oxygen gas) were placed into a cylindrical gold capsule and sintered for 10–30 min at 805–850 °C under a pressure of 2 GPa. To control the hole doping level, we have optimized the starting material, sintering condition, and annealing condition for each sample. Details are described in Supplementary Table 1 . Sample characterization The optimized nominal compositions to obtain single-phase materials were Hg 0.85 Ba 2 CaCu 2.15 O 6+δ for Hg1212 and Hg 0.75 Ba 2 Ca 2 Cu 3.25 O 8+δ for Hg1223. The analysed compositions determined by a scanning electron microscope (JSM-6701 F, JEOL) equipped with energy dispersive X-ray analyzer (XFlash detector 5030, Bruker AXS) were Hg:Ba:Ca:Cu=0.77:1.99:0.99:2.25 and 0.81:1.96:2.17:3.07, respectively. The powder X-ray diffraction patterns (RINT, Rigaku) confirmed the nearly single phase of Hg1212 and Hg1223. The scanning electron microscope images indicate that they are much denser than the samples prepared with the conventional silica-tube encapsulation method. The bulk superconductivity at ambient pressure was confirmed by dc-susceptibility measured with the field cooling procedure at 20 Oe (MPMS, Quantum Design) as well as by electrical resistivity (PPMS, Quantum Design). Resistivity measurement at high pressure The electrical resistivity at high pressure was measured using a cubic-anvil-type high-pressure apparatus with low-temperature cryostat (200 ton press, Rockgate Co.,). The samples with the four gold wires were placed in Teflon capsule with grease (Apiezon N) as a pressure-transmitting medium, and put in the gasket of MgO. To produce higher pressure, we use anvil tops with the sintered diamond. The anvils with the size of 4 × 4 mm 2 (sample size: 1.2 × 0.6 × 0.4 mm 3 ) and of 3 × 3 mm 2 (sample size: 0.8 × 0.4 × 0.3 mm 3 ) were used for the experiments up to 13 and 22 GPa, respectively. The sample temperature was determined with the Cernox resistance thermosensor on one of the anvil top. How to cite this article: Yamamoto, A. et al. High-pressure effects revisited for the cuprate superconductor family with highest critical temperature. Nat. Commun. 6:8990 doi: 10.1038/ncomms9990 (2015).